Direct chemical conversion of graphene to boron- and nitrogen- and carbon-containing atomic layers Graphene and hexagonal boron nitride are typical conductor and insulator, respectively, while their hybrids hexagonal boron carbonitride are promising as a semiconductor. Here we demonstrate a direct chemical conversion reaction, which systematically converts the hexagonal carbon lattice of graphene to boron nitride, making it possible to produce uniform boron nitride and boron carbonitride structures without disrupting the structural integrity of the original graphene templates. We synthesize high-quality atomic layer films with boron-, nitrogen- and carbon-containing atomic layers with full range of compositions. Using this approach, the electrical resistance, carrier mobilities and bandgaps of these atomic layers can be tuned from conductor to semiconductor to insulator. Combining this technique with lithography, local conversion could be realized at the nanometre scale, enabling the fabrication of in-plane atomic layer structures consisting of graphene, boron nitride and boron carbonitride. This is a step towards scalable synthesis of atomically thin two-dimensional integrated circuits. Graphene and hexagonal boron nitride (h-BN) are iso-structural two-dimensional materials with hexagonal honeycomb lattice atomic layers [1] , [2] . In spite of their structural similarities, the two materials are completely distinct electrically: graphene is a good conductor and h-BN is a good insulator [3] , [4] , [5] , [6] . Recently, several attempts have been made to build graphene devices on h-BN substrates to exploit their complementary properties [7] , [8] , [9] , [10] . Progress in this direction has been limited by difficulties in achieving scalable growth of uniform h-BN layers using chemical vapour deposition, a technique used to deposit high-quality graphene layers [11] , [12] , [13] , [14] , [15] , [16] , [17] , [18] , [19] . There have also been a few attempts to co-deposit graphene and h-BN domains to build hybridized two-dimensional boron carbonitride (h-BNC) atomic layers [10] , [11] , [12] , [13] , [14] , [15] , [16] , [17] , [18] , [19] , [20] , [21] , [22] . This coexistence of seamless graphene and h-BN domains inspires us to explore the synthesis of large area and high-quality h-BN atomic layers by substitutions of carbon atoms in graphene with boron and nitrogen. In this work, we report a topological substitution reaction that converts graphene to h-BNC and h-BN layers, which allows full control of composition, spatial variation and dimension of the G/h-BNC/h-BN interfaces and domains. We demonstrate good control of h-BN concentration from 0 to 100% and the compatibility of lithography technologies for lateral heterostructures, consisting of well-designed graphene, h-BNC and h-BN patterning. We provide a demonstration of tuning the conductivity, bandgap and on/off ratio of a ternary h-BNC 2D layer through a controllable transition from highly conductive graphene to semiconducting h-BNC and, finally, to insulating h-BN. To convert graphene to h-BN, solid boric acid powders are preloaded to the heating zone inside a quartz vacuum tube supplied with a flow of mixed ammonia and argon gas. Complete conversion from graphene to h-BN typically requires 2 h at 1,000 °C (see Methods). The proposed reaction formula and detailed nucleation energetics have been provided in the Supplementary Discussion . During the conversion, boron and nitrogen atoms gradually replace carbon atoms in the lattice until a highly conducting graphene film is completely converted into insulating h-BN atomic layers. If the conversion reaction is stopped in less than 2 h, partially converted h-BNC with variable BN concentration is obtained. The intermediate state in which B, C and N atoms coexist in the lattice exhibits the typical semiconducting properties of h-BNC films. Morphology and structure and composition characterization For the pristine graphene, converted h-BNC, and fully converted h-BN films shown in Fig. 1a–c , the carbon concentrations are 100%, 65% and 0%, respectively. The change in composition is directly reflected in the colour of the samples, changing from light purple to light blue in the optical micrographs [17] . The three structures have distinct Raman signatures ( Fig. 1d ) [23] , [24] , [25] . The high quality of the single-layered chemical vapour deposition (CVD) graphene is confirmed by the peak positions of the G and 2D bands (1,580 and 2,700 cm −1 ), the near absence of D band [26] , [27] , the ratio of 2D/G intensity (>4.0) and the scanning transmission electron microscopy (STEM) characterizations ( Fig. 2b and Supplementary Fig. 1 ). For the intermediate state h-BNC film, D mode (~1,350 cm −1 ) from graphene and E 2g mode (~1,370 cm −1 ) from h-BN contribute to a peak at 1,363 cm −1 ( Fig. 1e ). A shoulder of the G peak at 1,610 cm −1 is also observed [20] . For fully converted h-BN films, only the E 2g peak is detected at ~1,370 cm −1 and no 2D or G peaks are observed, demonstrating nearly complete substitution of carbon atoms [15] , [28] . The full width at half maximum of the E 2g peak in the h-BN is ~12 cm −1 , suggesting that the overall quality of the converted h-BN films is better than that of films made by direct CVD growth on copper foils (~16 cm −1 ) [15] and is comparable to that of mechanically exfoliated h-BN films (10~12 cm −1 ) [28] . X-ray photoelectron spectroscopy (XPS) was employed for chemical analysis of the pristine graphene template and the converted h-BNC and h-BN as illustrated in Fig. 1f–h . The calculated C, B and N atomic ratios for the three benchmarks are 100:0:0, 65:17:18 and 0:50:50, respectively. As the intensity of carbon peaked at 284 eV falls with lower carbon concentrations, the intensities of B (peaked at 190 eV) and N (peaked at 398 eV) rise. 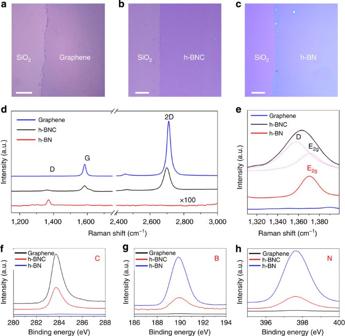Figure 1: Phase and composition characterization. (a–c) Optical images of graphene, h-BNC and h-BN, respectively. The colour of pristine graphene is light purple. B and N substitutions will change the colour from purple to blue for the fully converted h-BN. Scale bar for (a), (b) and (c) is 50, 20 and 20 μm, respectively. (d) and (e) Raman spectra of graphene, h-BNC and converted h-BN samples. There is no D peak in pristine graphene (blue). The h-BNC layers have D, G and 2D peaks, which contain signals from both graphene (D mode, ~1,350 cm−1) and h-BN (E2gmode, ~1,370 cm−1). The 2D and G peaks disappear in the fully converted h-BN. The peak at ~1,370 cm−1corresponds to theE2gvibration model of h-BN. (f–h) The 1 s core level XPS (X-ray photoelectron spectroscopy) spectra of carbon, boron and nitrogen, respectively. The black, red and blue lines are associated with graphene, h-BNC and h-BN, respectively. Figure 1: Phase and composition characterization. ( a – c ) Optical images of graphene, h-BNC and h-BN, respectively. The colour of pristine graphene is light purple. B and N substitutions will change the colour from purple to blue for the fully converted h-BN. Scale bar for ( a ), ( b ) and ( c ) is 50, 20 and 20 μm, respectively. ( d ) and ( e ) Raman spectra of graphene, h-BNC and converted h-BN samples. There is no D peak in pristine graphene (blue). The h-BNC layers have D, G and 2D peaks, which contain signals from both graphene (D mode, ~1,350 cm −1 ) and h-BN ( E 2g mode, ~1,370 cm −1 ). The 2D and G peaks disappear in the fully converted h-BN. The peak at ~1,370 cm −1 corresponds to the E 2g vibration model of h-BN. ( f – h ) The 1 s core level XPS (X-ray photoelectron spectroscopy) spectra of carbon, boron and nitrogen, respectively. The black, red and blue lines are associated with graphene, h-BNC and h-BN, respectively. 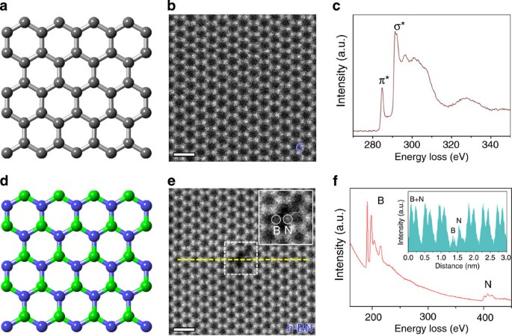Figure 2: Microstructure characterization of graphene and converted h-BN. (a) and (d) Schematic of graphene and h-BN. The carbon, nitrogen and boron atoms are in grey, blue and green, respectively. (b) An atomic resolution (Scanning transmission electron microscopy- annular dark field) STEM-ADF image of the graphene sample before conversion. (c) A corresponding EEL (electron energy loss) spectrum of graphene. (e) Atomic resolution STEM-ADF image of highly crystallized double layer h-BN converted from graphene. The darker area in the centre corresponds to single-layered h-BN, showing the presence of single-nitrogen atom (brighter one) and boron atom (darker one); this is further verified by intensity profile (inset inFig. 2f) of the atoms across the yellow-dashed line shown in (e). (f) A corresponding EEL spectra of the converted h-BN. The scale bar for both (b) and (e) is 0.5 nm. Full size image Figure 2: Microstructure characterization of graphene and converted h-BN. ( a ) and ( d ) Schematic of graphene and h-BN. The carbon, nitrogen and boron atoms are in grey, blue and green, respectively. ( b ) An atomic resolution (Scanning transmission electron microscopy- annular dark field) STEM-ADF image of the graphene sample before conversion. ( c ) A corresponding EEL (electron energy loss) spectrum of graphene. ( e ) Atomic resolution STEM-ADF image of highly crystallized double layer h-BN converted from graphene. The darker area in the centre corresponds to single-layered h-BN, showing the presence of single-nitrogen atom (brighter one) and boron atom (darker one); this is further verified by intensity profile (inset in Fig. 2f ) of the atoms across the yellow-dashed line shown in ( e ). ( f ) A corresponding EEL spectra of the converted h-BN. The scale bar for both ( b ) and ( e ) is 0.5 nm. Full size image Microstructure characterization The quality of prinstine graphene and fully converted h-BN films are further characterized by aberration-corrected STEM annular dark field (ADF) imaging and spectroscopy analysis. Schematic of graphene and fully converted h-BN are shown in Fig. 2a,d , while Fig. 2b,e present the atomic resolution STEM-ADF images of both samples. The darker area in the centre in Fig. 2e corresponds to single-layered h-BN, with the bottom layer of the double-layered converted h-BN partially peeled off by the electron beam, showing the clear presence of nitrogen atom (brighter one) and boron atoms (darker one) as marked with white circles in the inset. This is further demonstrated by image intensity profile (inset in Fig. 2f ) of the atoms across the yellow-dashed line, which shows signal corresponding to the superposition of boron and nitrogen atoms in the double-layer area and signal from single nitrogen and boron atoms in the single-layer area (dark region). Electron energy loss spectra (EELS) acquired from the regions shown in Fig. 2b,e further confirm that the graphene film was fully converted to h-BN ( Fig. 2c,f ). Most of the converted h-BN films were found to be single layer or bi layer by examining their edges, which is consistent with the atomic force microscopy (AFM) results ( Supplementary Fig. 2 ) [27] , [28] . The low magnification images of the graphene before and after conversion to h-BN can be found in Supplementary Fig. 1 . We noticed that, under low BN concentration, the h-BNC film looks uniform under optical and electron microscopes ( Supplementary Fig. 3 ). Increasing the reaction time and BN concentration will lead to the formation of h-BN nanodomains. The nanodomains in converted h-BNC are observed by the STEM-ADF imaging and elemental mapping ( Supplementary Fig. 4 ). At even higher BN concentration, the h-BN domains grow larger. Some of them merge into micro-scale h-BN islands, as identified by the Raman spectra ( Supplementary Fig. 5 ). We attribute this tendency to the lower interfacial energy induced by larger BN islands, whose interface lengths can be shorter than that of the separated BN domains, as will be discussed later. The detailed nucleation process of the BN domains is carefully studied by intensive density–functional theory (DFT) calculations. Our calculations propose a two-step mechanism for the conversion of graphene to h-BN, as illustrated in Fig. 3a–f by showing several typical snapshots through the conversion process. The first step refers to the inclusion of nitrogen or boron atoms in graphene, which energetically prefers to occur around structural imperfections in graphene, such as the defects, edges and functionalized carbon atoms by hydroxyl groups ( Supplementary Table 1 ). The high quality of graphene samples suggests that the functionalized carbon atoms should dominate the inclusion, especially considering that hydroxyl groups can be continuously introduced from the feedstock (the dissociation of boric acid) and silica substrates [29] , [30] , and extensively stick onto graphene [31] ; hence, only hydroxyls are shown in Fig. 3a . For the hydroxyls, we find that nitrogen atoms become highly favourable to substitute the functionalized carbon atoms while boron atoms remain unfavourable (see Supplementary Table 1 ), in agreement with our XPS analysis that only nitrogen can be found in graphene if the reaction was stopped at the very initial step ( Supplementary Fig. 3c ). Then, the second step is the nucleation of h-BN around the embedded nitrogen atoms. Indeed, the subsequent substitution of a boron atom or a BN pair becomes much easier around the embedded nitrogen atoms than in the bulk graphene area ( Supplementary Table 1 ). To simplify the discussion, we take the BNH 4 group as a representative source to investigate the thermodynamic growth of the BN domains in graphene. The substitution at each step can be either exothermic or endothermic ( Supplementary Fig. 11 and Supplementary Table 2 ), determined by the step-by-step increase in the length of BN–graphene interface. The optimal substitution pathway should always take a way that minimizes the total interface length, or with minimum number of B–C and N–C bonds. As a result, the initial tiny BN domains prefer to adopt a triangle shape [32] ( Fig. 3c,d ), at many random locations on the graphene template, rendering the h-BNC a spatially well-dispersed phase, but they could rapidly coarsen into an irregular shape by merging with neighbouring domains through continually supplying BN sources and long-time reaction ( Fig. 3e ); the latter is more frequent in our experiments under high BN concentrations. The merging of BN domains reduces the interface energy, thereby enhancing the substitution and expediting the conversion into h-BN ( Fig. 3f ). Total enthalpy of the reaction at our experimental condition, obtained from the formation enthalpy of products and reactants in the formula, amounts to the order of 275 kJ mol −1 ; thus, the BN conversion is an endothermic reaction that needs to be activated by the larger entropic contribution from the products at sufficiently high temperatures ( Supplementary Fig. 12a ). 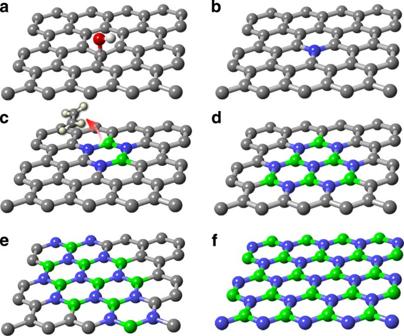Figure 3: Mechanism for the substitution from graphene to h-BN. The carbon, nitrogen, boron, oxygen and hydrogen atoms are in grey, blue, green, red and white, respectively. (a) CVD (chemical vapour deposition) graphene with adsorbed OH groups, introduced either from dissociated boric acid or intrinsic in graphene. (b) Substituting OH-adsorbed C atoms with N atoms. (c) Nucleation of BN domain from the embedded N atoms by BN substitutions, releasing a C2H4molecule at each step. (d) Initial BN domains prefer a triangle shape. (e) Further growth gets the BN domains in an irregular shape by merging with neighboring domains. (f) BN domains merge to achieve fully converted h-BN. Figure 3: Mechanism for the substitution from graphene to h-BN. The carbon, nitrogen, boron, oxygen and hydrogen atoms are in grey, blue, green, red and white, respectively. ( a ) CVD (chemical vapour deposition) graphene with adsorbed OH groups, introduced either from dissociated boric acid or intrinsic in graphene. ( b ) Substituting OH-adsorbed C atoms with N atoms. ( c ) Nucleation of BN domain from the embedded N atoms by BN substitutions, releasing a C 2 H 4 molecule at each step. ( d ) Initial BN domains prefer a triangle shape. ( e ) Further growth gets the BN domains in an irregular shape by merging with neighboring domains. ( f ) BN domains merge to achieve fully converted h-BN. Full size image This proposed mechanism can be supported by the complementary characterizations, such as XPS, Raman spectrum, optical and STEM imaging. The h-BNC films with well dispersed tiny BN domains are often observed at low BN concentrations. ( Supplementary Fig. 3 ). Under a high BN concentration, clear h-BN domains can be seen ( Supplementary Figs 4 and 5 ). The optical bandgaps (~2 eV) from graphene and h-BN (from 4 to 6 eV) can be derived from the UV spectra ( Supplementary Fig. 7f and Supplementary Note 1 ). Similar optical bandgap has also been found previously in heterogeneous h-BN/graphene film grown by using the CVD method [33] . These results suggest that our h-BNC film undergoes a change in morphology from spatially well-dispersed phase into in-plane hybrid structures rich in BN domains as the BN concentration increases, qualitatively consistent with our theoretical models. Decreasing the BN concentration reduces the insulating bandgap of h-BN domains, due to the enhanced conjugation effect of the surrounding graphene areas. In contrast, increasing the BN concentration shrinks the graphene size and endows the graphene areas with enhanced quantum confinement effect, which increases the band gap of graphene areas. Fractions of graphene strips can be found imbedded between h-BN domains from STEM imaging ( Supplementary Fig. 6 ). The bandgap evolution is confirmed by our first-principle calculations shown in Supplementary Fig. 12 , where the dependence of calculated bandgap of the h-BNC films on the h-BN concentration is consistent with our experimental measurements. Spatially controlled conversion can be achieved by using lithographically defined silica masks ( Fig. 4a–h ). First, we transfer pristine graphene onto a high-resistance silicon wafer as a media substrate ( Fig. 4a ). Then, a 50 nm layer of silica with predefined patterns is deposited atop the graphene by lithography process ( Fig. 4b ). After that, the whole chip is placed into a CVD furnace to apply the conversion reaction. Only the exposed graphene areas are converted while the areas covered by silica remain intact as graphene during the reaction ( Fig. 4c ). Once the conversion is complete, the silica mask is removed by HF solutions, and the films are transferred by PMMA onto other substrates ( Fig. 4d ). During conversion, the concentration of h-BN can be well controlled via the reaction time. A two-step template conversion process will convert pristine graphene into an in-plane graphene/h-BNC/h-BN heterostructure layer. Starting from the partially converted graphene/h-BNC ( Fig. 4e ), another mask is then fabricated to cover parts of the h-BNC region, and a second conversion undertaken to obtain h-BN area in the uncovered areas ( Fig. 4f,g ). Etching away the two masks using HF solutions, the preserved regions of graphene and h-BNC would serve as conducting and semiconducting regions embedded inside the passive h-BN lattices ( Fig. 4h ). Multiple conversion cycles further broaden the range of achievable complex heterostructure 2D layers containing graphene, h-BNC and h-BN layers. These patterns can be utilized in complex circuitry applications as shown in latter demos. 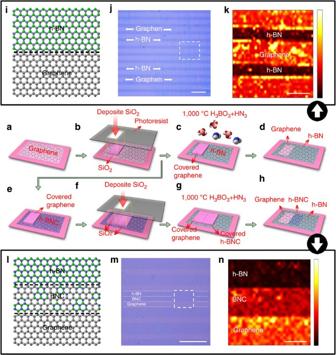Figure 4: Construction of graphene/h-BNC/h-BN in-plane 2D heterostructures. (a–d) Schematics of the spatially controlled conversion process of graphene into h-BN. (a) Transfer graphene onto a high-resistance intrinsic silicon wafer as a media substrate. (b) Deposit 50 nm SiO2with predefined patterns on top of the graphene. (c) Transfer the whole chip into a CVD (chemical vapour deposition) furnace for conversions. (d) Wash away the SiO2masks by buffered HF solutions and transfer the films via PMMA-KOH lift-offs onto other substrates. (a), (b) and (e–h) Two-step process that converts graphene into a graphene/h-BNC/h-BN heterostructure thin film. The first cycle (a,b) is identical to the steps explained previously, except that it stops at a partial-substitution intermediate state. (e) h-BNC surrounds a mask-protected graphene region. The second cycle starts with a new mask that protects regions where h-BNC needs to be preserved (f), and finishes the conversion until a perfect h-BN film is formed in the defined region (g,h). (i) Schematic of graphene/h-BN strip. (j) Optical image of graphene/h-BN alternative strips on SiO2substrate with a scale bar 10 μm. (k) Raman mapping at 2D peak (2,700 cm−1) of the marked area in (j) (scale bar, 5 μm). (l) Schematic showing the proposed atomic structure of a graphene/BNC/h-BN strip. (m) Optical image of graphene/h-BNC/h-BN alterative strips synthesized by this two-step conversion with a scale bar 40 μm. Raman mapping of the squared area from the 2D peak (2,700 cm−1) is shown in (n) (scale bar 10 μm). Figure 4i,j is the atomic schematic and an optical image of a graphene/h-BN alternative strip synthesized by the conversion method and transferred onto 285-nm SiO 2 substrate. The widths of the graphene and h-BN ribbons are ~6 and ~3 μm, respectively. Graphene and h-BN domains, distinguished by colour ( Fig. 4j ), are nicely integrated in this approach. Raman mapping ( Fig. 4k ) of the 2D peak (2,700 cm −1 ) was performed at the marked area in Fig. 4j . The bright regions indicate a high intensity of the 2D peak from graphene, while no 2D peak was found in the black regions where graphene was fully converted to h-BN [28] . Figure 4l shows the atomic structure model of a graphene/h-BNC/h-BN hybrid strip, which is exemplified in Fig. 4m by the optical image of a hybrid strip synthesized by the two-step template conversion process. The width of the strips is ~12 μm. In the Raman mapping of the highlighted area ( Fig. 4m,n ) with the 2D peak (2,700 cm −1 ), graphene, h-BNC and h-BN strips can be clearly seen as uniform domains with sharp interfaces between mask-defined regions, although the contrast between h-BN and h-BNC is relatively low in the optical image. Note that the h-BNC region exhibits a 2D Raman peak intensity between that of the surrounding graphene and h-BN material, consistent with our previous experiments. Complicated graphene/h-BN heterostructures, such as an Owl (the logo of Rice University), can be fabricated ( Supplementary Fig. 8a ), demonstrating that this versatile lithography-compatible conversion method can enable a much more complicated design. Furthermore, heterostructures with feature size less than 100 nm are demonstrated using the e-beam lithography-defined masks ( Supplementary Fig. 8b–d ). The as-prepared hybrid layers can be readily transferred onto flexible substrates, such as PDMS, showing promising application in flexible electronics ( Supplementary Fig. 8e ). Figure 4: Construction of graphene/h-BNC/h-BN in-plane 2D heterostructures. ( a – d ) Schematics of the spatially controlled conversion process of graphene into h-BN. ( a ) Transfer graphene onto a high-resistance intrinsic silicon wafer as a media substrate. ( b ) Deposit 50 nm SiO 2 with predefined patterns on top of the graphene. ( c ) Transfer the whole chip into a CVD (chemical vapour deposition) furnace for conversions. ( d ) Wash away the SiO 2 masks by buffered HF solutions and transfer the films via PMMA-KOH lift-offs onto other substrates. ( a ), ( b ) and ( e – h ) Two-step process that converts graphene into a graphene/h-BNC/h-BN heterostructure thin film. The first cycle ( a , b ) is identical to the steps explained previously, except that it stops at a partial-substitution intermediate state. ( e ) h-BNC surrounds a mask-protected graphene region. The second cycle starts with a new mask that protects regions where h-BNC needs to be preserved ( f ), and finishes the conversion until a perfect h-BN film is formed in the defined region ( g , h ). ( i ) Schematic of graphene/h-BN strip. ( j ) Optical image of graphene/h-BN alternative strips on SiO 2 substrate with a scale bar 10 μm. ( k ) Raman mapping at 2D peak (2,700 cm −1 ) of the marked area in ( j ) (scale bar, 5 μm). ( l ) Schematic showing the proposed atomic structure of a graphene/BNC/h-BN strip. ( m ) Optical image of graphene/h-BNC/h-BN alterative strips synthesized by this two-step conversion with a scale bar 40 μm. Raman mapping of the squared area from the 2D peak (2,700 cm −1 ) is shown in ( n ) (scale bar 10 μm). 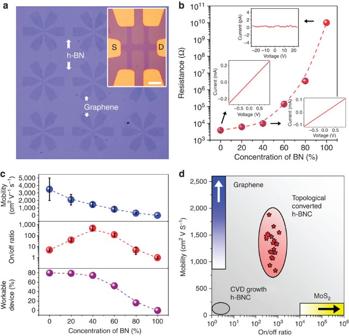Figure 5: Performance of h-BNC-based field-effect transistor. (a) Optical image of graphene/h-BN FET (field-effect transistor) arrays before depositing the contacts. Each FET consists of a 1 μm × 8 μm ribbon bridging six 100 μm × 100 μm graphene pads. Inset is the graphene ribbon under test and the scale bar is 2 μm. (b) Plot of the resistance versus the concentration of carbon showing the transition from a metal and semiconductor-like film to an insulating film. Insets: I-V curves from different samples as the arrow indicated. (c) Plot of the mobility, ON/OFF ratio and ratio of workable devices versus the carbon concentration. (d) Comparison of FET performance of h-BNC with other 2D materials such as graphene, transition metal dichalcogenides (TMDs) such as MoS2(ref.29). Twenty data points for the present study are shown in red stars. Full size image Figure 5 and Supplementary Fig. 9 present the electrical transport measurement of graphene and the h-BNC and h-BN films prepared by this conversion method. Graphene/h-BN FET arrays are shown in Fig. 5a before depositing contacts. The inset is a close-up of the source-drain carrier-transportation channel. The evolutions of electric parameters such as electric resistivity, mobility and on/off ratio of the FETs have been systematically measured and plotted in Fig. 5b,c . In a complete conversion cycle (atomic concentration of carbon decreases from 100% to 0), the resistivity of h-BNC first increases slightly and then goes up exponentially. An inverse tendency arises in the mobility. The source-drain current on/off ratio goes up initially followed by a decrease at ~60% carbon concentration. Such dependencies can be well correlated with the conversion picture we proposed above. In the case of slightly converted h-BNC, h-BN nucleates at the hydroxyl-functionalized carbon ( Fig. 3a–c ). The changes in the electric parameters imply a weak n -doping effect from the embedded N atoms or tiny h-BN domains ( Supplementary Fig. 9c ). If we keep the substitution reaction going, graphene will shrink into interconnected strips delimited by the h-BN domains ( Fig. 3d ). These quasi-one-dimensional strips provide not only paths for transport channels but also a narrow-bandgap corresponding to a high on/off ratio ( Supplementary Fig. 7f ). With increasing BN concentration, the enhanced confinement effect in the graphene channels will partly degrade the mobility in graphene. A good compromise between mobility and on/off ratio is observed in the h-BNC with ~60% carbon. Higher BN substitution will undermine the charge transport, as graphene channels are disconnected into nanodomains embedded in an h-BN matrix ( Fig. 3e ). The charge transport of this disordered system is likely dominated by a thermal-activated variable-rang hopping mechanism, leading to an exponential increase of the resistivity of the h-BNC films ( Fig. 5b ). Finally, the mobility and on/off ratio drop down to zero simultaneously when the graphene has been fully converted to h-BN. In other words, the h-BNC film undergoes the transition from metal-like, to semiconducting-like and to an insulating behaviour following the conversion. They are further supported by I–V curves (insets in Fig. 5b ). Low BN concentration leads to an Ohmic contact while source-drain current can be hardly detected at high concentration. It is important to note that, for high BN concentration, the ratio of workable devices markedly reduced to zero, an indication of percolation threshold at around 80% BN concentration. Figure 5: Performance of h-BNC-based field-effect transistor. ( a ) Optical image of graphene/h-BN FET (field-effect transistor) arrays before depositing the contacts. Each FET consists of a 1 μm × 8 μm ribbon bridging six 100 μm × 100 μm graphene pads. Inset is the graphene ribbon under test and the scale bar is 2 μm. ( b ) Plot of the resistance versus the concentration of carbon showing the transition from a metal and semiconductor-like film to an insulating film. Insets: I-V curves from different samples as the arrow indicated. ( c ) Plot of the mobility, ON/OFF ratio and ratio of workable devices versus the carbon concentration. ( d ) Comparison of FET performance of h-BNC with other 2D materials such as graphene, transition metal dichalcogenides (TMDs) such as MoS 2 (ref. 29 ). Twenty data points for the present study are shown in red stars. Full size image Most of the graphene FETs show mobilities in the range from 2,500 to 4,500 cm 2 V −1 s −1 ( Fig. 5c ), comparable to results reported for other CVD-grown polycrystalline graphene tested by back-gating configurations [34] , [35] , [36] . For the h-BNC films with 60% carbon, most of the FETs show mobilities in the range from 1,000 to 1,550 cm 2 V −1 s −1 and on/off ratio from 300 to 700. Compared with other 2D materials, our h-BNC films realized a good trade-off between high on/off ratio and acceptable carrier mobility ( Fig. 5d , red stars for our data; Supplementary Fig. 10 ). The reasonable mobility and on/off ratio in our h-BNC FET devices serve as an important step forwards for graphene-integrated circuitries [35] , [36] . In conclusion, we have demonstrated a novel synthesis method based on monolayer graphene template conversion, which enables the controlled conversion of conducting graphene into semiconducting ternary h-BNC and insulating h-BN, using a high-temperature topochemical conversion technique. The large-area films made by this method are highly crystalline and are able to preserve the electronic characteristics of graphene, h-BNC and h-BN in the same film with our template-based conversion method. First-principle calculations further reveal a novel reaction mechanism based on two-step nucleation of BN domains for this conversion. In addition, we have demonstrated functional devices based on the heterostructure layers made from conversion of graphene and transferred them onto multiple substrates. This work should allow exploration of new device architectures and synthesis strategies based on combining graphene, h-BN and h-BNC as the metal, semiconductor, insulator components of atomically thin circuit platforms. Material synthesis The substitution reaction is carried out in a quartz tube under high temperature. Graphene grown on copper foils is first transferred onto high-resistance intrinsic silicon substrates and then loaded into a vacuum quartz tube. The tube is pumped down to 60 mTorr with pure Argon flows for 15 min. Then the whole tube is heated up to 1,000 °C in 40 min and then kept at 1,000 °C when the reaction starts. Solid boric acid powder is preloaded in a boat inside the tube and heated up to 300–600 °C separately by heating wires surrounding the tube as a boron-releasing zone. Meanwhile 50 sccm ammonia gas flows as the source of nitrogen. Normally a reaction of 0.5 h leads to a 50% conversion, and a 2-h reaction will completely convert graphene to h-BN. After the reactions, the films are washed by 80 °C hot water twice to remove the boric acid or boron oxide residues on the surface. Finally, the film-on-silicon are coated by poly(methyl methacrylate) (PMMA) and then etching lifted-off by 10% potassium hydroxide (KOH) solution for further transferring. Characterization Atomic force microscopy (AFM, Agilent PicoScan 5500 and Veeco Digital Instrument Nanoscope IIIA) is used to determine the surface morphology of the samples. XPS (PHI Quantera XPS) is performed using monochromatic aluminium Kα X-rays. Raman spectroscopy (Renishaw inVia) is performed at 514.5 nm laser excitation at a power of 20 mW. High-resolution transmission electron microscopy (HRTEM, JEOL-2100) is employed to study the morphologies of h-BN and BNC layers at an accelerating voltage of 200 kV. The STEM experiments are performed with a Nion UltraSTEM-100, at an accelerating voltage of 60 kV. EELS are collected using a Gatan Enfina spectrometer, with an energy resolution of 0.6 eV. The convergence semi-angle for the incident probe is 31 mrad. ADF images are collected for a half-angle range of ~54–200 mrad. Device fabrication The films (graphene, h-BNC and h-BN) are transferred onto a highly doped silicon wafer with 300 nm SiO 2 and then metal electrodes (1.5 nm Ti/30 nm Au) were deposited on the graphene pads. The devices are annealed in vacuum at 300 °C for 0.5 h. All electrical measurements are carried out in the probe station along with an Agilent B1500A Semiconductor Device Analyzer under high vacuum (10 −5 torr). More than 40 electrical devices were fabricated based upon the same template conversion strategy with different heterostructure combinations and circuitry designs. Theoretical models All the theoretical calculations were performed with the Vienna Ab-initio Simulation Package [37] . The projector-augmented wave method for the core region and the generalized gradient approximation with the Perdew, Burke and Ernzerhof functional were employed. Kinetic energy cutoff of 500 eV was adopted in the plane-wave expansion. A 4 × 4 graphene supercell was used to simulate the incorporation of N atoms in graphene and the nucleation of BN domains. The Brillouin zone integration was sampled by 10 special k -points for structural optimization and energy calculations. The atomic positions and lattice constants are optimized by using the conjugate gradient method, and the maximum force allowed on each atom is less than 0.01 eV/Å. We also have chosen 2 × 6 and 10 × 2 k -point sampling for calculating the armchair and zigzag BN-graphene interface energy, respectively. For bandgap calculations, we used a 8 × 8 graphene supercell with varied BN concentrations and 45 special k -points for the Brillouin zone sampling. How to cite this article: Gong, Y. et al. Direct chemical conversion of graphene to boron- and nitrogen- and carbon-containing atomic layers. Nat. Commun. 5:3193 doi: 10.1038/ncomms4193 (2014).